The NMR structure of stomagen reveals the basis of stomatal density regulation by plant peptide hormones Stomatal development in plants is regulated by defensin-like secretory epidermal patterning factor (EPF) peptide hormones. Only one of these, stomagen, is a positive regulator, whereas EPF1, EPF2, and possibly others are negative regulators. Here we explore the structure–function relationships of EPFs, by integrating NMR and semi- in vitro stomagen experiments. We show that stomagen is composed of a loop and a scaffold containing three disulphide bonds. A mutant composed of the stomagen loop and the EPF2 scaffold positively regulates the stomatal density on Arabidopsis cotyledons. The reciprocal mutant composed of the EPF2 loop and the stomagen scaffold acts negatively. Deletion of the disulphide bond introduces unfolding and inactivity. Our results suggest that the loop confers the functional specificity of EPFs and that the scaffold is structurally required for their activity. This structural decomposition approach to elucidating the functional site could be adapted for the analysis of other cysteine-rich peptide families. Gas exchange in land plants is mediated by stomata, small pores formed by guard cells in the epidermal tissues of the surfaces of leaves and stems [1] , [2] . Stomatal development and density are negatively regulated by membrane proteins, including too many mouths (TMM) and ERECTA family of receptor-like kinases (ERf), which contain ER, ERL1 and ERL2 (refs 3 , 4 ). TMM and ERf receptors are thought to dimerize and function in a tissue-specific manner [4] , [5] . At least two possible ligands of the TMM–ERf complex, epidermal patterning factor 1 (EPF1) and EPF2, are negative regulators of stomatal density [3] , [6] , [7] , [8] , [9] . Extensive bioinformatic analyses of the Arabidopsis genome have revealed that several genes with unknown function are similar to EPF1 and EPF2 , and their products are considered to be members of the EPF family. These homologous peptides are defensin-like cysteine-rich secretory peptides and are classified as plant peptide hormones. Several EPF family members, including EPF1 and EPF2, function as the negative regulators of stomatal development. The functions of the other members remain unclear. Interestingly, it is currently known that stomagen (EPFL9) acts as a positive regulator [10] , [11] , [12] . One of the most intriguing questions in this area is how and why peptides from the same family can produce opposite effects on stomatal density. To understand the structure–function relationships of EPFs, we integrate NMR and semi- in vitro stomagen experiments. We solve the three-dimensional structure of stomagen by solution NMR. To the best of our knowledge, this is the first three-dimensional structural analysis of a plant peptide hormone. Furthermore, we find that the loop confers the functional specificity on EPFs and that the scaffold is structurally required for the activity of these peptides. Structure of stomagen Stable isotope-labelled NMR samples were prepared via a protein expression system using an inducible virus vector and suspension-cultured plant cells [13] . This NMR sample preparation method, which was originally developed by our group, has the advantage of allowing the expressed cysteine-rich proteins to fold with the proper formation of disulphide bonds [14] . We employed this method of sample preparation, as EPFs have six conserved cysteine residues ( Fig. 1a ). 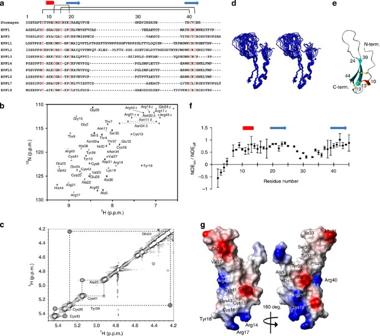Figure 1: Structure of stomagen. (a) The primary structures of the EPF family members fromArabidopsis. The sequence alignment was performed using ClustalW. The conserved cysteine residues are coloured red. Three pairs of stomagen disulphide bonds are indicated by lines. The cylinder and arrows denote helices and strands, respectively. (b) The1H-15N HSQC of stomagen. The asterisks represent peaks with very weak intensity. Five Arg side chain ɛ signals appear as folded peaks. (c) The downfield α1H-α1H region of the two-dimensional1H-1H NOESY spectrum for stomagen. The dotted lines indicate α1H-α1H NOE pairs within a β-sheet. Some peaks are labelled with their amino-acid type and residue number. (d) A stereoview of 20 NMR structures from stomagen. Only their backbones are depicted. (e) A ribbon model of stomagen. Three pairs of disulphide bonds are depicted in the ball-and-stick model. The secondary structural regions were estimated using MOLMOL. (f) The results of the {1H}-15N NOE experiments. The error bars show the s.d. (n=2). (g) The electrostatic potential distribution on the molecular surface of stomagen. Red, blue, and white indicate negative, positive, and hydrophobic, respectively. Some of the residues are labelled with amino-acid type and residue number. Figure 1b shows the 1 H- 15 N HSQC of stomagen. The narrow line shape and dispersion of signals suggest a single stable conformation. The downfield α 1 H-α 1 H region of the two-dimensional 1 H- 1 H nuclear Overhauser enhancement spectroscopy (NOESY) shown in Figure 1c suggests the existence of β-strands [15] . The results of the NMR-derived structural elucidation are presented in Figure 1d–g . The structural characteristics are summarized in Supplementary Table S1 . DALI ( http://ekhidna.biocenter.helsinki.fi/dali_server/ ) analysis suggested that stomagen adopts a novel folding pattern. Figure 1: Structure of stomagen. ( a ) The primary structures of the EPF family members from Arabidopsis . The sequence alignment was performed using ClustalW. The conserved cysteine residues are coloured red. Three pairs of stomagen disulphide bonds are indicated by lines. The cylinder and arrows denote helices and strands, respectively. ( b ) The 1 H- 15 N HSQC of stomagen. The asterisks represent peaks with very weak intensity. Five Arg side chain ɛ signals appear as folded peaks. ( c ) The downfield α 1 H-α 1 H region of the two-dimensional 1 H- 1 H NOESY spectrum for stomagen. The dotted lines indicate α 1 H-α 1 H NOE pairs within a β-sheet. Some peaks are labelled with their amino-acid type and residue number. ( d ) A stereoview of 20 NMR structures from stomagen. Only their backbones are depicted. ( e ) A ribbon model of stomagen. Three pairs of disulphide bonds are depicted in the ball-and-stick model. The secondary structural regions were estimated using MOLMOL. ( f ) The results of the { 1 H}- 15 N NOE experiments. The error bars show the s.d. ( n =2). ( g ) The electrostatic potential distribution on the molecular surface of stomagen. Red, blue, and white indicate negative, positive, and hydrophobic, respectively. Some of the residues are labelled with amino-acid type and residue number. Full size image In the structure of stomagen, two anti-parallel β-strands (residues 19–24 and 39–44) are connected by a 14-residue loop. The anti-parallel β-sheet is packed with the amino-terminal region, which contains a one-turn 3 10 -helix (residues 10–13), supported by three disulphide bonds, the locations of which (Cys8-Cys41, Cys13-Cys20, and Cys16-Cys43) were identical to those previously obtained by enzymatic digestion and mass spectrometry (MS) [11] . This stomagen core, consisting of the β-sheet and a one-turn 3 10 -helix, does not correspond to a single continuous stretch in the amino-acid sequence; it is separated into N- and carboxy-terminal regions (residues 8–24 and 39–44). These two regions, corresponding to the core, were found to cover relatively conserved regions in the amino-acid sequence alignment of the family ( Fig. 1a ). Six cysteine residues located in the core are particularly well conserved. In contrast to the core, the loop spans a largely divergent region in the amino-acid sequence alignment of the EPF family members. The loop region is inserted into the middle position of the amino-acid sequence ( Fig. 1a ). Unlike the scaffold, the 14-residue loop of stomagen has some flexibility as shown by the relatively small values in the { 1 H}- 15 N nuclear Overhauser effect (NOE) results ( Fig. 1f ). The electrostatic potential on the molecular surface of stomagen was calculated and is displayed in Figure 1g . One side of the molecular surface is relatively hydrophobic, and this side contains conserved cysteine residues in the scaffold. The surface of the stomagen loop has negatively charged regions, but no positively charged regions. As an extra structural analysis, the negative regulator EPF2 was subjected to MS and NMR. We attempted to prepare EPF2 without a tag sequence using the BY-2 cells, but the yield was too low. Thus, we added a 6×His-tag and a PreScission protease digestion site at the N terminus of EPF2. After the protease digestion and purification, the sample EPF2′ had two extra residues, Gly-Pro, at its N-terminal end as compared with the wild type, but it retained its activity ( Supplementary Fig. S1 ). Compared with stomagen, EPF2 itself contains two extra cysteine residues that are located in the loop region as shown in Figure 1a . MS of the products prepared by enzymatic digestion revealed that these cysteine residues in EPF2′ form a disulphide bond ( Supplementary Fig. S2a ). The one-dimensional 1 H-NMR of EPF2′ has lower-field shifted α 1 H resonances, suggesting that EPF2 has a β-sheet(s) ( Supplementary Fig. S2b ) [15] . These structural constraints suggest that EPF2 has a three-dimensional structure that is similar to that of stomagen. Subsequently, we used the structure of stomagen to attempt homology modelling of all of the other EPFs. These structure predictions suggested that all EPFs have a similar molecular fold ( Supplementary Fig. S3 ). Large amount of structural divergence among the EPFs was found in the loop, which, however, may correspond to functional differences among the peptides. Stomagen is antagonized by EPF2 Before beginning the semi- in vitro experiments using EPFs and the mutants, our negative control confirmed that stomatal development is not changed by external application of a peptide. We employed plectasin [16] , [17] , a peptide containing three disulphide bonds, whose function is not related to stomatal development. Plectasin was applied to 1DAG Arabidopsis plants to observe their capacity to induce stomata formation. The negative control peptide was found not to affect the stomatal development ( Fig. 2a ). Moreover, plectasin did not influence the function of stomagen ( Fig. 2b ). These plectasin results support the reliability of our semi- in vitro experiments. 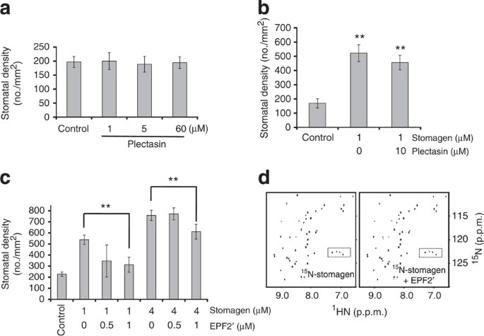Figure 2: Stomagen competes with EPF2. (a) The effect of plectasin, a negative control, on the stomatal density ofArabidopsiscotyledons. The error bars show s.d. (n>5). (b) The effect of plectasin in the presence of stomagen. Plectasin does not compete with stomagen. The error bars show s.d. (n>5). **P<0.01 versus the controls by the Wilcoxon two-sample test. No significant difference was seen between the middle and the right. (c) The dose-dependent effect of stomagen and EPF2′ on the stomatal density ofArabidopsiscotyledons. The error bars show s.d. (n>8). **P<0.01 by the Wilcoxon two-sample test. (d) The1H-15N HSQC of15N-labelled stomagen in the absence (left) and presence (right) of unlabelled EPF2′. The resonance assignments are shown inSupplementary Figure S1. The fold-back peaks of the Arg side chains are shown in the boxes. Figure 2: Stomagen competes with EPF2. ( a ) The effect of plectasin, a negative control, on the stomatal density of Arabidopsis cotyledons. The error bars show s.d. ( n >5). ( b ) The effect of plectasin in the presence of stomagen. Plectasin does not compete with stomagen. The error bars show s.d. ( n >5). ** P <0.01 versus the controls by the Wilcoxon two-sample test. No significant difference was seen between the middle and the right. ( c ) The dose-dependent effect of stomagen and EPF2′ on the stomatal density of Arabidopsis cotyledons. The error bars show s.d. ( n >8). ** P <0.01 by the Wilcoxon two-sample test. ( d ) The 1 H- 15 N HSQC of 15 N-labelled stomagen in the absence (left) and presence (right) of unlabelled EPF2′. The resonance assignments are shown in Supplementary Figure S1 . The fold-back peaks of the Arg side chains are shown in the boxes. Full size image For the biological experiments, chemically synthesized stomagen was refolded, and EPF2′ was prepared as described. Both stomagen and EPF2′ were applied to 1DAG Arabidopsis plants to observe their capacity to induce stomata formation. The addition of stomagen increased the stomatal density, but it was decreased by EPF2′ ( Fig. 2c ; Supplementary Fig. S1 ). Moreover, the effect of EPF2′ was evident even in the presence of stomagen and was concentration dependent ( Fig. 2c ). Figure 2c clearly indicates that the differences in the amount of stomagen and EPF2′ determine their overall effect on stomatal development. We also observed the 1 H- 15 N HSQC spectra of 15 N-labelled stomagen in the absence and presence of EPF2′ ( Fig. 2d ). No significant difference was found between these two spectra. The NMR results indicate that stomagen does not interact with EPF2′ in vitro . These results suggest that the functional competition observed in Figure 2c was not caused by a direct interaction between stomagen and EPF2′. Role of the disulphide bonds We next examined the role of the disulphide bonds using a chemically synthesized stomagen mutant in which two of the six conserved cysteine residues were replaced by serine residues ( Fig. 3a ). We also prepared a chemically synthesized stomagen mutant, C/S, in which all the cysteine residues were replaced by serine residues ( Fig. 3a ). The downfield-shifted α 1 H signals resonating from the residues forming β-sheet disappeared in the one-dimensional 1 H-NMR spectra of the mutants ( Fig. 3b ). The NMR results strongly suggest that the introduction of these mutations disrupted the overall structure [15] . For the C/S mutant in particular, the disappearance of the downfield-shifted α 1 H signals showed a complete loss of the β-sheet structure ( Fig. 3b ). 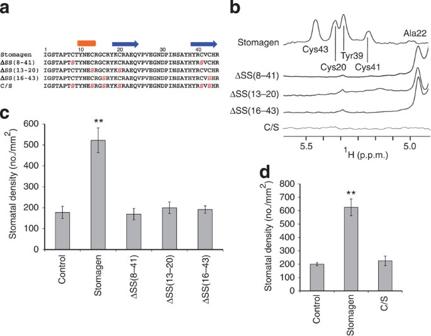Figure 3: The structure and function are lost when the conserved Cys residues are replaced. (a) The amino-acid sequences of stomagen and the ΔSS and C/S mutants. The red letters indicate the mutation points. (b) The downfield α1H region of the1H-NMR spectra of stomagen (top) and the mutants. (c,d) The effect of the mutant peptides on the stomatal density ofArabidopsiscotyledons; the concentration of the stomagen and the mutants is 3 μM. The error bars show s.d. (n>8). **P<0.01 versus the controls by the Wilcoxon two-sample test. Figure 3: The structure and function are lost when the conserved Cys residues are replaced. ( a ) The amino-acid sequences of stomagen and the ΔSS and C/S mutants. The red letters indicate the mutation points. ( b ) The downfield α 1 H region of the 1 H-NMR spectra of stomagen (top) and the mutants. ( c , d ) The effect of the mutant peptides on the stomatal density of Arabidopsis cotyledons; the concentration of the stomagen and the mutants is 3 μM. The error bars show s.d. ( n >8). ** P <0.01 versus the controls by the Wilcoxon two-sample test. Full size image Although all of the ΔSS mutants were expected to form two disulphide bonds, enzymatic digestion and MS analyses showed that an incorrect disulphide bond was formed ( Supplementary Figs S4-S6 and Supplementary Tables S2-S4 ). For example, Δ(8–41) was expected to have two disulphide bonds at Cys13–Cys20 and Cys16–43, but our results showed that a disulphide bond at Cys20–Cys43 was formed, but the other two cysteine residues, Cys13 and Cy43, did not form a disulphide bond. Therefore, the incorrect formation of the disulphide bonds results in an improper conformation ( Fig. 3b ). A similar irregular disulphide bond formation was observed for the other two variants; for ΔSS(13–20) and ΔSS(16–43), only the Cys8–Cys16 and Cys20–Cys41 disulphide bonds, respectively, were formed. These results strongly suggest that all three pairs of disulphide bonds are necessary to form the consensus scaffold. Semi- in vitro experiments showed that mutations eliminating one or three disulphide bonds had no effect on the stomatal density ( Fig. 3c,d ). It is likely that the lack of disulphide bonds made it difficult for the resulting unstructured mutants to adopt an active conformation. We also examined short peptides corresponding to the complete or partial regions of the stomagen loop. These peptides had no effect on stomatal density ( Supplementary Fig. S7 ). These findings suggest that the small peptides corresponding to the stomagen loop are not significant enough to have any effect. Therefore, we focused our attention on the loop's context in the entire peptide. The loop confers the peptide's function We designed and prepared two kinds of loop-swapped mutants to measure their activity ( Fig. 4a ). One was EPF2′-St, which was composed of the EPF2 scaffold and the stomagen loop; the other was the reciprocal chimera, St′-EPF2, which was composed of the stomagen scaffold and the EPF2 loop. Similar to EPF2′, both of these peptides had two extra residues at the N terminus after the enzymatic digestion during the sample preparation ( Fig. 4a ). EPF2′-St was found to increase the stomatal density of Arabidopsis cotyledons in a concentration-dependent manner ( Fig. 4b,c ). Thus, the data indicate that EPF2′-St acts as a positive regulator, even though EPF2 itself is a negative regulator of stomatal development. Unlike EPF2′-St, the reciprocal chimera, St′-EPF2, decreased the stomatal density of the Arabidopsis cotyledons, although the effect seemed to be slightly weaker than that of EPF2′ ( Fig. 4d,e ). These loop-swapped mutants clearly demonstrated that the loop confers the function to the EPF peptides. 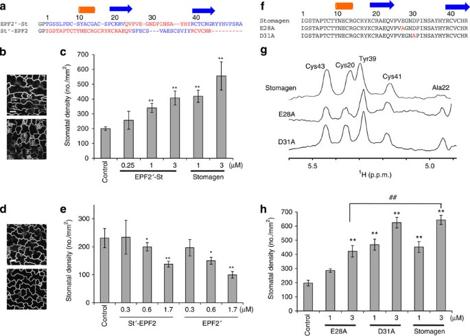Figure 4: Swapping and point mutations reveal the functional importance of the loop. (a) Amino-acid sequences of the stomagen mutants (EPF2′-St and St′-EPF2) used in these experiments. The red and blue letters indicate the amino-acid sequences of stomagen and EPF2, respectively. The first two residues, GP, are the extra residues that remain after the protease digestion during purification. (b) Confocal images of the abaxial epidermis ofA. thalianacotyledons that were treated with no peptide (top) or the EPF2′-St (bottom). The scale bar in the image indicates 50 μm. (c) The stomatal density in the presence of the EPF2′-St or stomagen at different concentrations. The error bars show s.d. (n>8). **P<0.01 versus the controls analysed by the Wilcoxon two-sample test. (d) Confocal images of the abaxial epidermis ofA. thalianacotyledons that were treated with no peptide (top) or the St′-EPF2 (bottom). The scale bar in the image indicates 50 μm. (e) The stomatal density in the presence of the St′-EPF2 or stomagen at different concentrations. The error bars show s.d. (n>8), *P<0.05 and **P<0.01, respectively, versus the controls in the Wilcoxon two-sample test. (f) The amino-acid sequences of stomagen and the Ala mutants. The red letters indicate the mutation points. (g) Downfield α1H region of1H-NMR spectra of stomagen (top) and the Ala mutants (others). (h) Effect of the mutant peptides on the stomatal density ofArabidopsiscotyledons. The error bars show s.d. (n>8). **P<0.01 versus the controls in the Wilcoxon two-sample test.##P<0.01 between the two indicated treatments in the Wilcoxon two-sample test. Figure 4: Swapping and point mutations reveal the functional importance of the loop. ( a ) Amino-acid sequences of the stomagen mutants (EPF2′-St and St′-EPF2) used in these experiments. The red and blue letters indicate the amino-acid sequences of stomagen and EPF2, respectively. The first two residues, GP, are the extra residues that remain after the protease digestion during purification. ( b ) Confocal images of the abaxial epidermis of A. thaliana cotyledons that were treated with no peptide (top) or the EPF2′-St (bottom). The scale bar in the image indicates 50 μm. ( c ) The stomatal density in the presence of the EPF2′-St or stomagen at different concentrations. The error bars show s.d. ( n >8). ** P <0.01 versus the controls analysed by the Wilcoxon two-sample test. ( d ) Confocal images of the abaxial epidermis of A. thaliana cotyledons that were treated with no peptide (top) or the St′-EPF2 (bottom). The scale bar in the image indicates 50 μm. ( e ) The stomatal density in the presence of the St′-EPF2 or stomagen at different concentrations. The error bars show s.d. ( n >8), * P <0.05 and ** P <0.01, respectively, versus the controls in the Wilcoxon two-sample test. ( f ) The amino-acid sequences of stomagen and the Ala mutants. The red letters indicate the mutation points. ( g ) Downfield α 1 H region of 1 H-NMR spectra of stomagen (top) and the Ala mutants (others). ( h ) Effect of the mutant peptides on the stomatal density of Arabidopsis cotyledons. The error bars show s.d. ( n >8). ** P <0.01 versus the controls in the Wilcoxon two-sample test. ## P <0.01 between the two indicated treatments in the Wilcoxon two-sample test. Full size image Finally, we focused our attention on the charge distribution on the stomagen loop surface. As shown in Figure 1g , two negatively charged regions formed by the solvent-exposed charged residues E28 and D31 are found on the functional loop surface. We performed mutation experiments in which these charged residues were individually replaced with alanine ( Fig. 4f ). The 1 H-NMR data confirmed that these mutations did not disturb the stomagen conformation ( Fig. 4g ). The semi- in vitro experiments showed that the E28A mutant displays weaker activity than the wild type stomagen, whereas the D31A mutant functions similarly to stomagen ( Fig. 4h ). Thus, we deduced that E28 contributes to stomagen activity, and that D31 does not. In this paper, we reported the three-dimensional structure of stomagen and used it to explore the structure–function relationships of the EPF family. We found that stomagen is composed of a loop and a scaffold, and semi- in vitro experiments clearly demonstrated that the loop confers function. Stomagen activity is antagonized by that of EPF2, providing a clue to the interaction between them, but the present NMR study suggested that stomagen does not interact with EPF2. Therefore, three possible explanations for the antagonistic action observed here arise. The first is that these peptides share an identical binding site for their common target and that their binding occurs in a competitive manner. A second option is that they interact with different sites of the common target; in this case, the initial binding may influence subsequent interactions. The final scenario is that they bind different targets. It is possible that there are extra, as yet unidentified, factors involved in this regulatory system. The NMR-derived structure showed that the functional loop of stomagen is relatively hydrophobic. Moreover, it was found that E28 that is located in the loop is required for full stomagen activity. As shown in Figure 1g , E28 is located on the side of the hydrophobic molecular surface containing the conserved cysteine residues in the consensus scaffold. If this surface directly interacts with the target, then the target presumably has a hydrophobic molecular surface containing positive charges. It is interesting to note that both TMM and ERfs, which likely form a heterodimer that is thought to be a target of stomagen, are predicted to have hydrophobic leucine-rich repeats in their outer-membrane domains [4] , [5] . It is known that leucine-rich repeats is often employed for molecular recognition [18] . The scaffold of stomagen is stabilized by three disulphide bonds and represents a novel fold in the structural classification database. The mutation experiments suggested that the three pairs of disulphide bonds formed by the six cysteine residues are necessary for stabilizing the consensus scaffold among the EPFs. Therefore, these cysteine residues should have been conserved during molecular evolution. By contrast, it is expected that mutations could be more easily introduced into the loop, leading to differentiation into many types of EPF peptides with various activities. The existence of many EPF family peptides with different activities would be essential for achieving the subtle and complicated regulation of stomatal density. One way to understand their functional harmonization may be to analyse their spatiotemporal expression profile. Further structural and functional analyses focusing on the C-terminal region of EPFs, which is another divergent region in the amino-aid sequence alignment, may also suggest some biological significance. Similar to EPFs, defensin-like cysteine-rich families such as SCRLs and LUREs have been identified recently as regulators of biological processes in plants [19] , [20] . Although their three-dimensional structures seem to be different from those of the stomagen fold, a similar structural decomposition approach could be helpful for learning about their functional sites. Dividing their amino-acid sequences into a region containing the family-consensus disulphide bonds and other less conserved regions could help to delimit their functional site(s). Peptides The stomagen, EPF2 and stomagen mutants used in this study were overexpressed in BY-2 cells unless otherwise indicated. The chemically synthesized peptides were purchased (Promega). Vector construction and peptide expression The primers used in this study are summarized in Supplementary Table S5 . The tomato mosaic virus-based expression vector, used for expressing stomagen, EPF2′, EPF2′-St and St′-EPF2, was constructed by using pBICER8-C0.3-HuIFN-γ-SRz [21] to replace the IFN gene with complementary DNAs encoding for stomagen, EPF2′, EPF2′-St or St′-EPF2. The EPF2′, EPF2′-St and St′-EPF2 had a tag sequence (HHHHHHLEVLFQGP) at their N-terminal ends for purification purposes. These cDNAs were amplified by PCR using the primers shown in Supplementary Table S5 . The constructs were introduced into transgenic BY-2 cells expressing the β-oestrogen-activatable transcription factor XVE. Each transgenic BY2 suspension-cultured cell lines was maintained at 26 °C, transferring 1 ml of the saturated suspension cultured to 100 ml of fresh Murashige and SKoog's liquid medium each week. Expression of these peptides was induced by addition of 10 μM 17 β-estradiol to the culture, 2 days after subculture. The tag sequences in the EPF2′-St secreted to the medium were digested by host proteases. Expression of stable isotope-labelled peptides Unlabelled, 15 N-labelled and 13 C- and 15 N-labelled samples were prepared for NMR study. To prepare uniform 15 N-labelled NMR samples, stable isotope-labelled K 15 NO 3 and 15 NH 4 15 NO 3 were dissolved into the medium, at concentrations of 1,900 and 1,650 mg l −1 , respectively, to serve as nitrogen sources [14] . Similarly, uniform 13 C-labelled sucrose was employed for 13 C-labelling. Other protocol for peptide expression was identical to that described above. Peptide purification The culture medium of the BY-2 cells expressing stomagen or EPF2′-St was ultracentrifuged at 1,000,000 g for 30 min and the supernatant was filtered through a 0.22 μm filter. The filtrate was applied to a reverse-phase HPLC column. After washing the column with a solution of 5% methanol and 0.5% TFA, an elution was performed with a methanol linear gradient (5–90%). The EPF2′ and St′-EPF2 was purified by affinity chromatography using a Hi-Trap chelating column followed by PreScission protease digestion. The protease and copurified host proteins were removed by glutathione S -transferase and Ni 2+ affinity columns. The purity of the samples was verified by SDS–PAGE and matrix-assisted laser desorption/ionization–time-of-flight mass spectrometry (MALDI–TOF-MS) (Voyager DE RP, Applied Biosystems). Refolding of the synthesized peptides Chemically synthesized stomagen were dissolved in 20 mM Tris–HCl, pH 8.8, and 50 mM NaCl. The sample solution was dialysed for 1 day at 4 °C against 0.5 mM glutathione and 200 mM L -arginine at pH 8.0. Then, the sample solution was dialysed three times against the adequate buffer for NMR or biological assay. Enzymatic digestion and MS of variants Each refolded peptide (30 μg) was lyophilized and dissolved in 40 μl of 8 M urea solution. These samples were then diluted with 400 μl of ammonium bicarbonate. Two micrograms of trypsin was added to each solution. The samples were incubated at 37 °C for 1 h and subsequently kept at room temperature for 1 h. Additionally, all of the samples were incubated at 4 °C for 6 h, either without or with DTT (5 μl for each 50 μl sample). Each digested peptide solution was purified and concentrated with a ZipTip C18 pipette tip (Millipore). These purified samples were mixed with an á-cyano-4-hydroxycinnamic acid matrix (in 50% acetonitrile with 0.1% TFA) and analysed on a MALDI-TOF-MS. Semi- in vitro assay The sample peptides were applied to 1DAG Arabidopsis thaliana Columbia-0 plants that had germinated in a B5 sterilized liquid medium. After three further days of incubation at 22 °C, the stomatal densities on the abaxial cotyledons were determined by inspection with a confocal microscope [12] . NMR samples All of the samples for the NMR study were dissolved into H 2 O/D 2 O=90/10 or 100% D 2 O containing 100 mM KCl at pH 5.8 (by direct pH meter reading). The sample concentration was ∼ 0.6 mM. NMR experiments and structure calculation All the NMR data were obtained on a Bruker AVANCE III 800 spectrometer equipped with a TCI cryogenic triple-resonance probe. The sample temperature was kept at 25 °C during the NMR experiments. The 1 H- 15 N HSQC, HNCO, HNCA, CBCA(CO)NH, and HNCACB were measured for backbone resonance assignment [22] , [23] , [24] , [25] . The HCCH-TOCSY (mixing time=23 ms) and 2D-TOCSY (mixing time=43 ms) were measured for side-chain resonance assignment [26] , [27] . 2D-NOESY (mixing time=80, 150 and 200 ms) and 15 N-edited NOESY (mixing time=80, 150 and 200 ms) were used to obtain the distance information [28] , [29] . The NMR data processing and analysis were performed using NMRPipe [30] . The analyses of the NMR spectra were performed using NMRView [31] and Sparky [32] . The NOEs, H-bonds based on the secondary structure, and dihedral angles in the secondary structures were used as the constraints for the structure calculation [33] . The structures were calculated using a sa.inp protocol in Xplor-NIH 2.26. A total of 690 NMR-derived constraints were obtained for the calculation. One hundred structures were calculated and 93 structures were deemed acceptable and without large violations ( Supplementary Table S1 ). Finally, the 20 structures with the lowest energy terms were selected and analysed. Structural quality was examined with PROCHECK [34] . All of the structural figures were generated using MOLMOL [35] . Homology modelling of other EPFs Because stomagen has a new type of fold, no similar structure had been deposited in the protein data bank. Because of the lack of an adequate template, the structure prediction websites linked to the database, such as Swiss-Prot, did not work well. Therefore, we used the structure of stomagen as the template, and the homology modelling was performed using the Modeller [36] , [37] , [38] , [39] and EasyModeller [40] programs on a personal computer. The conserved disulphide bonds remained fixed during the model building steps. Accession codes: The coordinate and chemical shift data were deposited in Protein Data Bank (Code: 2LIY ) and Biological Magnetic Resonance Data Bank (accession number: 11452), respectively. How to cite this article: Ohki, S. et al . The NMR structure of stomagen reveals the basis of stomatal density regulation by plant peptide hormones. Nat. Commun. 2:512 doi: 10.1038/ncomms1520 (2011).